Efficient solar water splitting by enhanced charge separation in a bismuth vanadate-silicon tandem photoelectrode Metal oxides are generally very stable in aqueous solutions and cheap, but their photochemical activity is usually limited by poor charge carrier separation. Here we show that this problem can be solved by introducing a gradient dopant concentration in the metal oxide film, thereby creating a distributed n + –n homojunction. This concept is demonstrated with a low-cost, spray-deposited and non-porous tungsten-doped bismuth vanadate photoanode in which carrier-separation efficiencies of up to 80% are achieved. By combining this state-of-the-art photoanode with an earth-abundant cobalt phosphate water-oxidation catalyst and a double- or single-junction amorphous Si solar cell in a tandem configuration, stable short-circuit water-splitting photocurrents of ~4 and 3 mA cm −2 , respectively, are achieved under 1 sun illumination. The 4 mA cm −2 photocurrent corresponds to a solar-to-hydrogen efficiency of 4.9%, which is the highest efficiency yet reported for a stand-alone water-splitting device based on a metal oxide photoanode. The development of solar water-splitting devices has been the focus of many researchers recently, because the realization of such devices provides an attractive route to convert sunlight into a chemical fuel in the form of hydrogen. Various tandem device configurations have been proposed, but the optimal design is still not clear [1] , [2] , [3] , [4] , [5] , [6] . One approach is to combine a solar cell with hydrogen and oxygen evolution catalysts. Devices with a solar-to-hydrogen (STH) efficiency of up to 2.5%, consisting of triple-junction amorphous silicon (3-jn a-Si) solar cells with hydrogen and oxygen evolution catalysts, were demonstrated as early as 20 years ago [5] , [6] . Based on the same concept, along with a breakthrough in the development of cobalt-based water-oxidation catalysts that work in near-neutral pH conditions [7] , Nocera and coworkers [8] demonstrated an improved STH efficiency of up to 4.7%. In all these cases, however, a photovoltaic (PV) cell with a rather high open-circuit voltage ( V oc >1.6 V) is needed to provide the thermodynamic potential for water splitting (1.23 V) plus the necessary overpotentials [9] . As the catalytic efficiency of the cobalt-based water-oxidation catalyst is already close to one [10] , any major efficiency improvements for this approach would require PV devices with higher operating voltages and currents. Considering that 3-jn a-Si solar cells are already quite complex, the feasibility of such a strategy is doubtful. Alternatively, one may replace one or two of the p–i–n junctions in a 3-jn a-Si solar cell with a single semiconducting metal oxide film. Metal oxides are generally stable in water and form a junction at the semiconductor/water interface, providing an elegant, simple and low-cost alternative to the p–i–n junction. Moreover, the larger bandgap of the metal oxide allows better use of the solar spectrum and can lead to higher efficiencies than a pure Si-based device. Miller et al. [4] have argued that such a ‘hybrid photoelectrode’ has the potential of achieving 16% STH efficiency. By combining a double-junction a-Si (2-jn a-Si) solar cell and a tungsten trioxide (WO 3 ) photoanode, they predicted a 2.2% STH efficiency and demonstrated a practical efficiency of 0.6%. Later, they improved the performance and demonstrated an efficiency of 3% [11] . In a similar concept, Brillet et al. [12] recently showed a 3.1% efficient system by combining a WO 3 photoanode and a dye-sensitized solar cell (DSSC). The rather modest efficiency of these efforts is a result of the low conduction band energy and the large bandgap of the WO 3 photoanode. To achieve the 10% STH efficiency target, a metal oxide with a maximum bandgap of 2.3–2.4 eV is required. Here we demonstrate a solar water-splitting device based on the combination of a W-doped BiVO 4 photoanode and a 2-jn a-Si solar cell. By introducing a gradient in the dopant profile, it is possible to create a distributed n + –n homojunction in BiVO 4 that greatly enhances the charge-separation efficiency, thereby effectively removing its main performance bottleneck. In combination with an efficient earth-abundant water-oxidation catalyst and an a-Si solar cell connected in tandem, this provides a new and highly effective strategy for developing efficient solar water-splitting devices. Gradient W-doped BiVO 4 homojunction In the monoclinic phase, BiVO 4 is an n-type photoactive semiconductor with a bandgap of 2.4 eV [13] , [14] , [15] , with a conduction band positioned close to the hydrogen evolution potential [16] . In the last 2 years, the photoelectrochemical performance of BiVO 4 has been significantly improved [17] , [18] , [19] , [20] , [21] . This has been largely due to the development of novel water-oxidation catalysts based on, for example, cobalt- and iron oxyhydroxide-based materials [7] , [18] . As a result, the best-performing BiVO 4 photoanodes are no longer limited by slow water-oxidation kinetics, but by poor carrier separation due to slow electron transport in BiVO 4 (ref. 17 ). Although the introduction of a donor-type dopant, such as W or Mo [19] , [20] , [21] , [22] , can increase the conductivity of BiVO 4 , this is by itself not sufficient because of the low intrinsic mobility of BiVO 4 (ref. 23 ). As one cannot easily modify the intrinsic mobility, a different strategy is needed to improve the carrier separation. To achieve good carrier separation in a semiconductor photoanode, the presence of a built-in electric field (band bending) is required. One of the most common ways to enhance band bending in a photoanode is by combining it with another semiconductor, creating a heterojunction [16] , [23] , [24] . It is, however, not always trivial to find materials with suitably aligned energy levels, and a clean heterostructure can be difficult to synthesize. Improper growth conditions may lead to the presence of large amounts of defects at the interface that might act as carrier traps and recombination centres [25] , [26] . Moreover, the high carrier concentration in doped BiVO 4 —which is needed to address its low intrinsic mobility—reduces the extent of the space charge region to just a few nanometres. To avoid these complications, we introduce a step in the dopant concentration to distribute the band bending over a larger region in the bulk of the sample, and thereby improve the carrier separation. The principle is illustrated in Fig. 1 . Undoped BiVO 4 is an n-type semiconductor, and donor-doping it with tungsten (W) raises its Fermi level. When W-doped and undoped BiVO 4 are brought into contact, the Fermi energy levels equilibrate by electron transfer from the W-doped part to the undoped part of the material. A modest depletion layer at the interface between W-doped and undoped BiVO 4 is then formed that enhances charge separation. In contrast to a heterojunction, the synthesis of a homojunction is usually trivial, and the extent of the band bending can be tailored by simply varying the dopant concentration. 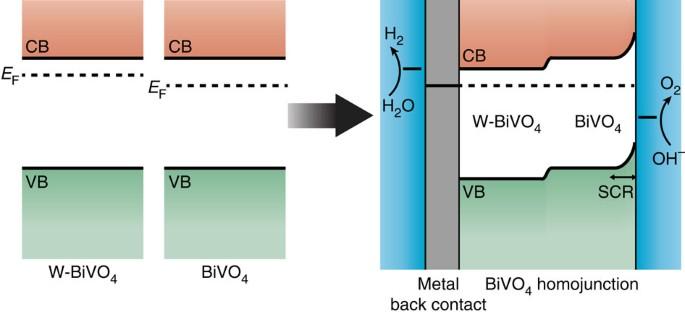Figure 1: The formation of a BiVO4homojunction. Energy band schematic of W-doped BiVO4(W-BiVO4) and BiVO4, showing the valence band (VB), conduction band (CB) and the Fermi level energy (EF). When they are brought into contact, the Fermi level energy will equilibrate and additional band bending is introduced, on top of the existing one at the space charge region (SCR), forming a BiVO4homojunction. Figure 1: The formation of a BiVO 4 homojunction. Energy band schematic of W-doped BiVO 4 (W-BiVO 4 ) and BiVO 4 , showing the valence band (VB), conduction band (CB) and the Fermi level energy ( E F ). When they are brought into contact, the Fermi level energy will equilibrate and additional band bending is introduced, on top of the existing one at the space charge region (SCR), forming a BiVO 4 homojunction. Full size image The use of a homojunction to enhance carrier separation is a well-established concept in semiconductor physics. Both p–n homojunctions and homojunctions in which a gradient in the composition causes a corresponding gradient in the band gap (for example, In x Ga 1− x N, CdS 1− x Se x and Ga 1− x Al x As) are well-known methods to enhance bulk carrier separation. The physical principles are, however, somewhat different than the one we employ here. Our approach resembles the Back Surface Field method [27] , which is usually implemented as a p + –p junction near the back contact of a-Si or GaAs solar cell that reflects the minority carriers and minimizes recombination at the interface. The main difference is that our distributed n + –n homojunction enhances charge separation throughout the bulk of the material, not just at the interface. To the best of our knowledge, this concept has not yet been reported before. This is perhaps not as surprising as it seems, because this approach only makes sense for very highly doped semiconductors, a class of materials that is not typically used as a light absorber. To demonstrate this concept, ~200-nm thick BiVO 4 photoanode samples with different dopant profiles were synthesized by spray pyrolysis. We first compare a 1% W-doped BiVO 4 sample ( Fig. 2a ) with a homojunction of 1% W-doped/undoped BiVO 4 ( Fig. 2b ). Because of the additional band bending in the W:BiVO 4 homojunction, we expect an enhanced carrier separation. To quantify the carrier-separation efficiency, we use an elegant formulation first reported by Dotan et al. 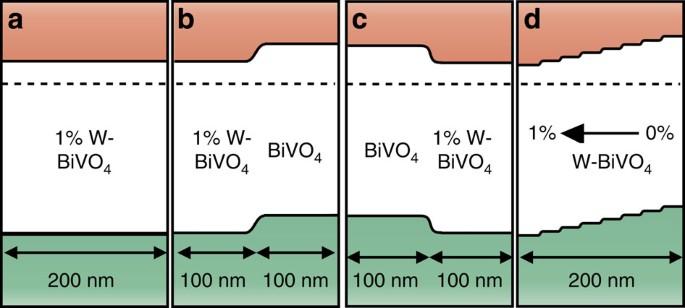Figure 2: Band diagram schematic of the BiVO4samples. (a) 1% W-doped BiVO4(W-BiVO4), (b) W:BiVO4homojunction, (c) W:BiVO4reverse homojunction and (d) gradient-doped W:BiVO4. In all cases, the light enters from the right-hand side (through the electrolyte), and the FTO back contact is situated on the left. The space charge region at the semiconductor/electrolyte interface is not depicted for clarity. [28] : Figure 2: Band diagram schematic of the BiVO 4 samples. ( a ) 1% W-doped BiVO 4 (W-BiVO 4 ), ( b ) W:BiVO 4 homojunction, ( c ) W:BiVO 4 reverse homojunction and ( d ) gradient-doped W:BiVO 4 . In all cases, the light enters from the right-hand side (through the electrolyte), and the FTO back contact is situated on the left. The space charge region at the semiconductor/electrolyte interface is not depicted for clarity. Full size image where J ph is the total photocurrent density, J abs is the photon-absorption rate expressed as current density, η sep is the carrier-separation efficiency and η cat is the catalytic efficiency for water oxidation. The differences between the internal/external quantum efficiencies and the carrier-separation efficiency are explained in the Supplementary Note 1 . When a highly effective hole scavenger such as hydrogen peroxide (H 2 O 2 ) is added into the electrolyte, the catalytic efficiency can be assumed to be ~100% ( η cat =1) (refs 28 , 29 , 30 ). This allows one to directly calculate the separation and oxidation efficiencies from the measured photocurrents with and without H 2 O 2 : and (ref. 28 ). As expected, the carrier-separation efficiency of the W:BiVO 4 homojunction is higher than that of the W:BiVO 4 reference sample ( Fig. 3 ), indicating that the dopant concentration difference can indeed be used to create additional band bending and thus improve carrier separation. 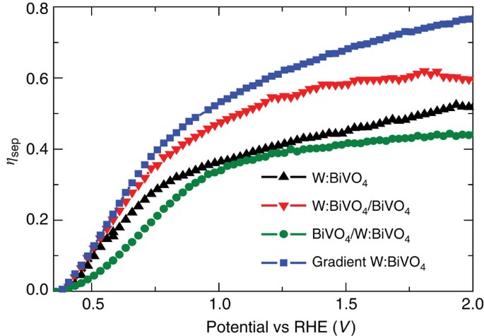Figure 3: Carrier separation efficiency. Carrier-separation efficiency (ηsep) as a function of applied potential for 1% W-doped BiVO4(black triangle), W:BiVO4homojunction (red inverted triangle), W:BiVO4reverse homojunction (green circle) and gradient-doped W:BiVO4(blue square). Figure 3: Carrier separation efficiency. Carrier-separation efficiency ( η sep ) as a function of applied potential for 1% W-doped BiVO 4 (black triangle), W:BiVO 4 homojunction (red inverted triangle), W:BiVO 4 reverse homojunction (green circle) and gradient-doped W:BiVO 4 (blue square). Full size image To confirm the presence of the homojunction, we also prepared a reverse homojunction in which the W-doped side is now closest to the electrolyte ( Fig. 2c ). In this case, the band bending is present in the opposite direction and should act as a barrier for carrier separation. As shown in Fig. 3 , the carrier-separation efficiency indeed decreases and is even lower than that of the homogeneously doped reference sample. The decrease is, however, not as big as one might have expected; the reason is that this barrier is actually small enough for a few electrons to overcome thermally (see Supplementary Note 2 ). Nevertheless, this observation provides compelling support for our claim that the improvement in carrier-separation efficiency is caused by the additional band bending at the W:BiVO 4 /BiVO 4 homojunction interface. To fully leverage this effect, we synthesized a BiVO 4 photoanode with a 10-step gradient in W doping, starting from 1% W at the interface with the back contact to 0% W at the semiconductor/electrolyte interface ( Fig. 2d ). This extends the presence of band bending over the entire thickness of the photoanode. As a result, we find that the carrier-separation efficiency increases to ~60% at 1.23 V versus reversible hydrogen electrode (RHE) ( Fig. 3 , blue curve), compared with ~38% for homogeneously doped BiVO 4 . This 1.6 × improvement shows that a gradient in dopant concentration can be used as a simple, yet highly effective, method to enhance the carrier separation in highly doped semiconductor photoelectrodes. To further correlate the improvement in carrier-separation efficiency to the band bending in the film, we measure the change in open circuit potential (ΔOCP) upon AM1.5 illumination. At this illumination intensity, the number of carriers is sufficiently high to achieve a maximum flattening of the energy bands ( Supplementary Fig. S1 ). The amount of band flattening depends on both the built-in potential and the extent of recombination in the film. The ΔOCP value systematically increases when going from the reference sample→W:BiVO 4 homojunction sample→gradient-doped W:BiVO 4 sample ( Supplementary Fig. S2a ). Because the total built-in potential is the same for all samples ( Supplementary Fig. S2b,c ), the increase in ΔOCP clearly indicates that there is less recombination in this sample. This is consistent with the larger number of space charge regions, one for each step in the concentration ( Fig. 2d ), and the improved spatial distribution of the electric field over the film thickness. We also observe in Supplementary Fig. S2 that the initial ΔOCP for the reverse homojunction is smaller than that of the reference sample, and it eventually reaches the same value. This indicates that there is initially more recombination, as indeed expected, and that the final ΔOCP is determined by the potential drop in the space charge region in the 1% W-doped BiVO 4 next to the semiconductor/electrolyte interface. Finally, we note that the appearance, optical absorption, morphology and crystal structure of all samples are the same, that is, these properties are not affected by the distribution of the tungsten dopant and cannot explain the improved charge separation ( Supplementary Figs S3–S6 ). Under AM1.5 illumination, the gradient-doped W:BiVO 4 shows a photocurrent of ~1.1 mA cm −2 at 1.23 V versus RHE ( Fig. 4 , solid black curve). To improve the oxygen evolution kinetics, we electrodeposited a 30-nm thick cobalt phosphate (Co-Pi) catalyst layer. Based on our previous study [17] , this thickness gives an optimum catalytic improvement for BiVO 4 and ensures that >90% of the incident light reaches the BiVO 4 . This results in an approximately threefold improvement of the AM1.5 photocurrent, up to 3 mA cm −2 at 1.23 V versus RHE ( Fig. 4 , red curve). To improve the performance even further, we replace the standard TEC-15 substrate with a textured Asahi VU-type conducting glass substrate. As a result of higher absorption and effective surface area ( Supplementary Fig. S7 ), this further improves the AM1.5 photocurrent to ~3.6 mA cm −2 at 1.23 V versus RHE ( Fig. 4 , blue curve). This is the highest photocurrent ever reported for BiVO 4 , and represents a ~1.6 × improvement compared with the best Co-Pi-catalysed W:BiVO 4 photoanode reported previously [10] . It also exceeds the highest AM1.5 photocurrents reported at this potential for α-Fe 2 O 3 (ref. 31 ) and WO 3 (ref. 32 ) (both ~3 mA cm −2 ) by a considerable margin, which firmly establishes BiVO 4 as the new leading performer among oxide photoanodes. 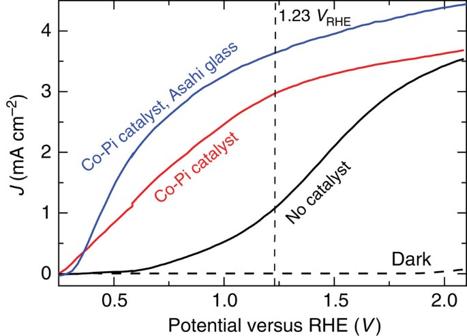Figure 4: Cyclic voltammetry. Three-electrode AM1.5 photocurrent versus voltage (J–V) curve of uncatalysed gradient-doped W:BiVO4on TEC-15 (black), Co-Pi-catalysed gradient-doped W:BiVO4on TEC-15 (red) and on Asahi conducting glass (blue). The dark current is shown as a dashed black curve. The electrolyte used is 0.1 M potassium phosphate buffer at pH ~7.3. Figure 4: Cyclic voltammetry. Three-electrode AM1.5 photocurrent versus voltage ( J – V ) curve of uncatalysed gradient-doped W:BiVO 4 on TEC-15 (black), Co-Pi-catalysed gradient-doped W:BiVO 4 on TEC-15 (red) and on Asahi conducting glass (blue). The dark current is shown as a dashed black curve. The electrolyte used is 0.1 M potassium phosphate buffer at pH ~7.3. Full size image Hybrid photoelectrode To fabricate a complete device for solar water splitting that does not depend on an externally applied bias potential, we combined the state-of-the-art Co-Pi–W:BiVO 4 photoanode with a 2-jn a-Si superstrate PV cell placed behind the photoelectochemical (PEC) cell, as shown in Fig. 5 . Details of the PV cell and a photograph of the hybrid device are shown in Supplementary Figs S8 and S9 , respectively. In this tandem configuration, photons with energies less than the bandgap of the BiVO 4 are absorbed by the a-Si/a-Si PV structure ( Supplementary Fig. S11 ). Figure 6a shows the J – V curve of the 2-jn a-Si solar cell (black curve) that has been optimized—by tuning the thickness of the individual absorber layers—to match the two-electrode J – V curve of the state-of-the-art BiVO 4 photoanode (blue curve). 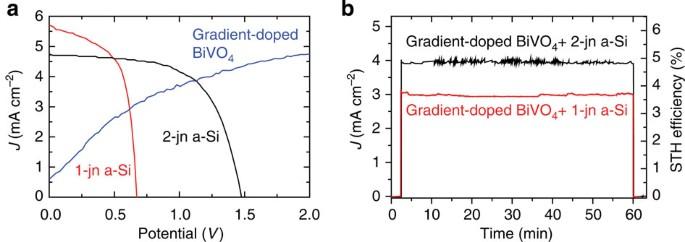Figure 6: PEC performance of the hybrid photoelectrode. (a) Two-electrode AM1.5J–Vcurve of Co-Pi-catalysed gradient-doped BiVO4on Asahi transparent conducting oxide glass (gradient-doped BiVO4, blue curve). Also shown are theJ–Vcurves of 2-jn a-Si (black) and single-junction a-Si (red) solar cells placed behind the Co-Pi–BiVO4:W photoanode. The intersection of the BiVO4curve with either one of the a-Si curves indicates the operating point of the combined water-splitting device. (b) Current versus time for the Co-Pi–BiVO4:W/2-jn a-Si device and the Co-Pi–BiVO4:W/1-jn a-Si device in the hybrid photoelectrode configuration under AM1.5 illumination. The electrolyte used is 0.1 M potassium phosphate buffer at pH ~7.3. It should be noted that the J – V curve of the BiVO 4 photoanode in the two-electrode measurement of Fig. 6a shows slightly larger photocurrents than the curve in the three-electrode measurement of Fig. 4 ; the reason for this is explained in the Supplementary Note 3 . Based on the intersection of the two curves in Fig. 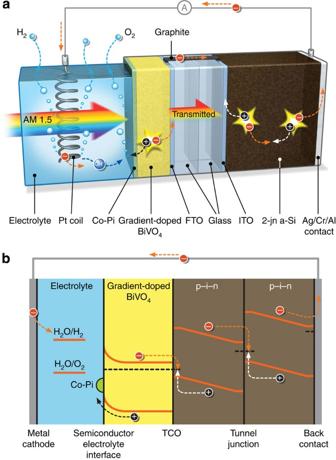6a , an operating photocurrent of ~4 mA cm −2 is predicted for the integrated device. Figure 5: Hybrid photoelectrode. (a) Schematic diagram of the combined device of gradient-doped W:BiVO4and a-Si solar cell. (b) The corresponding band diagram of the hybrid photoelectrode device. ITO, tin-doped indium oxide; TCO, transparent conducting oxide. Figure 5: Hybrid photoelectrode. ( a ) Schematic diagram of the combined device of gradient-doped W:BiVO 4 and a-Si solar cell. ( b ) The corresponding band diagram of the hybrid photoelectrode device. ITO, tin-doped indium oxide; TCO, transparent conducting oxide. Full size image Figure 6: PEC performance of the hybrid photoelectrode. ( a ) Two-electrode AM1.5 J – V curve of Co-Pi-catalysed gradient-doped BiVO 4 on Asahi transparent conducting oxide glass (gradient-doped BiVO 4 , blue curve). Also shown are the J – V curves of 2-jn a-Si (black) and single-junction a-Si (red) solar cells placed behind the Co-Pi–BiVO 4 :W photoanode. The intersection of the BiVO 4 curve with either one of the a-Si curves indicates the operating point of the combined water-splitting device. ( b ) Current versus time for the Co-Pi–BiVO 4 :W/2-jn a-Si device and the Co-Pi–BiVO 4 :W/1-jn a-Si device in the hybrid photoelectrode configuration under AM1.5 illumination. The electrolyte used is 0.1 M potassium phosphate buffer at pH ~7.3. Full size image Figure 6b shows the AM1.5 photocurrent of the tandem PEC/PV device as a function of time. A stable photocurrent of ~4 mA cm −2 is achieved, which indeed corresponds to the working point of the J – V curve of Fig. 6a . Because the Faradaic efficiency of this system is 100% [20] , this corresponds to a STH conversion efficiency of ~4.9%, which is a 60% improvement compared with a similar device based on 2-jn a-Si / WO 3 reported by Miller et al. [4] , [11] . This efficiency is also superior to the 4.7% efficiency benchmark recently reported by Nocera and coworkers [8] , who were the first to report on the remarkable efficiency of the Co-Pi catalyst under pH-neutral conditions [7] . Although the water-oxidation catalyst that we use is the same, the 2-jn a-Si cell we use is much easier to fabricate than the triple-junction device reported by Reece et al. [8] To illustrate that the gradient-doped W:BiVO 4 generates part of the total photovoltage, the same AM1.5 photocurrent measurement was done with the 2-jn a-Si cell connected to a Co-Pi film deposited directly on fluorine-doped tin oxide (FTO) substrate (that is, without the BiVO 4 ). This results in a much lower photocurrent of ~1.5 mA cm −2 ( Supplementary Fig. S12 ), despite the fact that the Co-Pi/FTO electrode transmits a much larger part of the solar spectrum to the underlying 2-jn a-Si cell. This confirms that BiVO 4 provides additional electromotive driving force and that the Co-Pi–W:BiVO 4 /2-jn a-Si device is effectively a triple-junction system. An important advantage of using BiVO 4 instead of other metal oxides in the hybrid photoelectrode configuration is its higher conduction band energy. This translates into a modest photocurrent onset potential of +0.25 V versus RHE for BiVO 4 ( Fig. 4 ). For comparison, the photocurrent onset potentials for Fe 2 O 3 and WO 3 are +0.8 V versus RHE and +0.5 V versus RHE, respectively [32] , [33] . A lower onset potential directly relaxes the demand on the voltage provided by the PV cell and allows simpler and cheaper designs to be pursued. In fact, based on the intersection of the J – V curves, Fig. 6a suggests that photocurrent of 3 mA cm −2 can be achieved by combining the gradient-doped BiVO 4 with a single-junction a-Si solar cell ( Supplementary Fig. S8 ). This photocurrent is indeed obtained for an actual hybrid one-junction a-Si (1-jn a-Si)/Co-Pi–W:BiVO 4 device, as shown by the red curve in Fig. 6b . This relatively simple device shows a 3.6% STH efficiency with no sign of degradation within the 1-h measurement period. Another advantage of BiVO 4 is that high photocurrrents can be obtained for compact, thin film electrodes. In contrast, many other metal oxide photoelectrodes require highly optimized nanostructures to ensure that the minority carriers can reach the surface before they recombine or to avoid limitations due to slow surface reaction kinetics. Apart from the fact that they are easier to make, compact films also avoid potential mass transport problems that may arise due to gas bubble formation within mesoporous structures. Another advantage of non-porous electrodes is the limited amount of light scattering, which may prevent the low-energy photons from reaching the bottom cell. This was found to be a problem for tandem water-splitting devices based on nanostructured α-Fe 2 O 3 electrodes and DSSCs. These devices showed efficiencies of 1.36%, significantly below the predicted value of 3.3% [34] . Recently, the EPFL group solved these problems and reported STH efficiencies of 1.17% and 3.1% for stand-alone water-splitting devices based on nanostructured Fe 2 O 3 /DSSC and WO 3 /DSSC devices, respectively [12] . The shapes of the J – V curves of the a-Si/BiVO 4 devices shown in Fig. 6a indicate that little or no further improvement can be gained from improving the currents delivered by the silicon PV devices. Instead, future efforts should initially focus on improving the light absorption and carrier-separation efficiency in BiVO 4 . The current films absorb 75% of the incident AM1.5 light with hν > E g , whereas the carrier-separation efficiency is still <60% at the working point of the device—despite the large improvement by the gradient-doping profile. Based on the near-unity internal quantum efficiencies that can be achieved in this defect-tolerant material [10] , addressing these remaining issues may lead to AM1.5 photocurrents that are close to the theoretical value of 7.5 mA cm −2 . Further development of these efficient hybrid photoelectrodes into practical solar water-splitting modules requires several engineering challenges to be solved. Although the near-neutral pH of the electrolyte solution ensures that the BiVO 4 is photochemically stable [35] , proton transport is markedly slower than in strongly alkaline or acidic electrolytes. The consequences of such mass transport limitations are clearly illustrated by the results of Nocera and coworkers [8] , who showed that their solar-to-H 2 efficiency dropped from 4.7 to 2.5% when changing the cell configuration from two electrodes that face each other, to a configuration in which H 2 and O 2 evolve from opposite sides of an ‘artificial leaf’. The design of new device architectures that efficiently manage proton transport and avoid local pH changes in near-neutral solutions thus represents an important challenge for future photoelectrochemical energy-conversion studies. Once the optimal device configuration is chosen, the evolved gasses need to be transported away efficiently without the risk of mixing. Finally, the platinum counter electrode that we used here for convenience needs to be replaced by an earth-abundant alternative. Such alternatives, for example, in the form of NiMo(Zn) [8] , CoMo or NiFeMo alloys [36] , are already available and show high activities at modest overpotentials. In summary, we have shown that the poor carrier-separation efficiency in BiVO 4 photoanode can be overcome by implementing a multi-step gradient in the tungsten dopant concentration, resulting in the formation of a series of homojunctions in the bulk of the material. A 10-step gradient-doped Co-Pi-catalysed W:BiVO 4 photoanode generates an AM1.5 photocurrent of 3.6 mA cm −2 at 1.23 V versus RHE, representing a ~60% improvement over the same electrode with a homogeneous W-dopant concentration [10] . Combining this electrode with a 2-jn a-Si solar cell results in a water-splitting device with a ~4.9% STH efficiency. This represents a significant improvement over other oxide-based tandem devices that have been reported recently [11] , [12] and sets a new performance benchmark for hybrid photoelectrodes for water splitting. It also exceeds the efficiency of more complicated silicon-based PEC devices based on three p–i–n junctions [8] . Replacing one p–i–n stack (and the accompanying tunnel junction) with a single wide-bandgap metal oxide absorber, both simplifies the design and increases the efficiency that can be achieved. Further improvements require a better utilization of the solar spectrum by BiVO 4 , especially for wavelengths close to the band edge, and plasmonic- and/or resonance-enhanced optical absorption [37] , [38] seem promising routes to achieve this. Finally, the distributed n + –n homojunction concept represents a generally applicable strategy for improving carrier separation in any high-donor density photoelectrode material. Combined with the hybrid photoelectrode concept, this offers new pathways towards low-cost, efficient devices for solar hydrogen generation. Synthesis Dense thin films of BiVO 4 were prepared using spray pyrolysis. The preparation of the precursor solution and the spray pyrolysis setup are described elsewhere [10] , [17] . The spray deposition rate is ~1 nm per cycle. The 1% W-doped BiVO 4 sample was prepared by spraying 200 cycles of the BiVO 4 precursor solution containing 1 at% of W. The W:BiVO 4 homojunction was prepared by spraying 100 cycles of the BiVO 4 precursor solution containing 1 at% of W, followed by 100 cycles of the BiVO 4 precursor solution. This sequence was reversed for the deposition of the W:BiVO 4 reverse homojunction. To deposit the gradient-doped W:BiVO 4 , the concentration of W in the BiVO 4 precursor solution was changed in step every 20 cycles, starting from 1 to 0 at%. Before every deposition, ~80 nm of SnO 2 layer was deposited onto FTO substrate to prevent recombination of electrons and holes at the FTO/BiVO 4 interface [39] . The substrates used are either TEC-15 (15 Ω per square; Hartford Glass Co.) or Asahi VU-type (8 Ω/sq; Asahi Glass Co.) FTO-coated glass. After the deposition, all samples were annealed for 2 h at 450 o C in air to further improve the crystallinity. A 30-nm Co-Pi catalyst was electrodeposited according to the recipe from Kanan and Nocera [7] . The electrodeposition was performed at a constant voltage of 1.7 V versus RHE for 15 min. Care was taken to always keep the electrodeposited Co-Pi layer wet, as intermediate drying of the Co-Pi was found to adversely affect the stability. The 2-jn a-Si and 1-jn a-Si solar cells were deposited on textured Asahi VU-type substrates. For the 2-jn a-Si, boron-doped hydrogenated a-Si (a-SiC:H) carbide, intrinsic a-SiC:H and a-Si:H are used as p layers, buffer layers and i layers, respectively. The n layer of the top cell is a single layer of phosphorus-doped microcrystalline silicon oxide, whereas the n layer of the bottom cell is a double layer of phosphorus-doped microcrystalline silicon oxide and phosphorus-doped a-SiC:H. For the 1-jn a-Si solar cell, boron-doped a-SiC:H carbide is used as the p layer, whereas the i layer and n layer are intrinsic a-SiC:H (a-Si:H) and phosphorus-doped a-SiC:H, respectively. These various silicon alloys were deposited using the radio-frequency plasma-enhanced chemical vapour deposition technique in a multi-chamber tool. After the deposition of the silicon thin films, the front contact (300 nm Al) and the back contact (100 nm Ag, 30 nm Cr and 400 nm Al) were deposited by a rotating Provac evaporator. The metal back contacts have a diameter of 7 mm and a size of 1 × 1 cm for the 2-jn a-Si and 1-jn a-Si, respectively. The gradient-doped BiVO 4 photoanode and the a-Si solar cell were then assembled to fabricate an integrated ‘hybrid photoelectrode’ device (as shown in Fig. 5 and Supplementary Fig. S9 ) using an ultra-clear two-component epoxy adhesive (Loctite Hysol 3430), pasted on the glass side of each device. Photoelectrochemical characterization Photoelectrochemical characterization was carried out in an aqueous 0.1 M potassium phosphate electrolyte solution (pH ~7.3). The potential of the working electrode was controlled by a potentiostat (EG&G PAR 283). In three-electrode measurements, a coiled Pt wire and an Ag/AgCl electrode (XR300, saturated KCl and AgCl solution; Radiometer Analytical) were used as the counter and reference electrodes, respectively. Two-electrode measurements were conducted by connecting the working electrode lead of the potentiostat to the BiVO 4 photoanode and the reference and counter electrode leads of the potentiostat to the coiled Pt wire. Cyclic voltammetry measurements were performed with a scan rate of 50 mV s −1 . White light photocurrent measurements were performed under simulated AM1.5 solar illumination (100 mW cm −2 ) with a Newport Sol3A Class AAA solar simulator (type 94023 A-SR3). Electrical contact to the sample was made using a silver wire and a graphite paste. A Keithley 2001 multimeter was used as the ammeter in the current versus time measurement of the tandem device. Physical characterization Structural analysis was performed with a Bruker D8 Advance X-ray diffractometer (Co-K α , λ =0.178897, nm) equipped with a LynxEye detector in the Bragg–Brentano configuration. Scanning electron micrographs were taken with JEOL JSM 6500F scanning electron microscope at an accelerating voltage of 15 kV. The ultraviolet-visible absorption was measured with a Perkin Elmer Lambda 900 spectrometer. How to cite this article: Abdi, F. F. et al. Efficient solar water splitting by enhanced charge separation in a bismuth vanadate-silicon tandem photoelectrode. Nat. Commun. 4:2195 doi: 10.1038/ncomms3195 (2013).